Surface passivated halide perovskite single-crystal for efficient photoelectrochemical synthesis of dimethoxydihydrofuran Halide perovskite single-crystals have recently been widely highlighted to possess high light harvesting capability and superior charge transport behaviour, which further enable their attractive performance in photovoltaics. However, their application in photoelectrochemical cells has not yet been reported. Here, a methylammonium lead bromide MAPbBr 3 single-crystal thin film is reported as a photoanode with potential application in photoelectrochemical organic synthesis, 2,5-dimethoxy-2,5-dihydrofuran. Depositing an ultrathin Al 2 O 3 layer is found to effectively passivate perovskite surface defects. Thus, the nearly 5-fold increase in photoelectrochemical performance with the saturated current being increased from 1.2 to 5.5 mA cm −2 is mainly attributed to suppressed trap-assisted recombination for MAPbBr 3 single-crystal thin film/Al 2 O 3 . In addition, Ti 3+ -species-rich titanium deposition has been introduced not only as a protective film but also as a catalytic layer to further advance performance and stability. As an encouraging result, the photoelectrochemical performance and stability of MAPbBr 3 single-crystal thin film/Al 2 O 3 /Ti-based photoanode have been significantly improved for 6 h continuous dimethoxydihydrofuran evolution test with a high Faraday efficiency of 93%. In the past decade, the vast latent capacity of halide perovskites in solar energy utilization has been reported; e.g., perovskite solar cells showed a power conversion efficiency of 25.5% [1] . In addition to solar-to-electricity conversion, the high light harvesting capability, superior carrier transport, and suitable band position of halide perovskites motivate the wide applications of these materials in photocatalysis and photoelectrochemical (PEC) fields [2] , [3] , [4] , [5] , [6] . Compared to particulate photocatalytic systems, PEC systems feature semiconductor photocatalysts and external biases and thereby exhibit significant advantages in high-efficiency charge separation and collection as well as easy catalyst recycling [7] . Recently, halide perovskite polycrystalline thin films (PCTFs) have been exploited for PEC water splitting and CO 2 reduction [8] , [9] , [10] , [11] , [12] , [13] , [14] , [15] , [16] , [17] . The use of organic solvent instead of water not only is expected to improve the stability of photoelectrode [18] , but also enables a broader set of organic synthesis reactions, achieving higher Faradaic efficiency and value-added chemicals [19] , [20] , [21] , [22] , [23] , [24] , [25] . Compared to PCTFs, perovskite single-crystal thin films (SCTFs) inherit the advantages of both polycrystalline films and bulk single crystals [26] , such as low trap-state densities, long carrier diffusion lengths, well-defined thicknesses and, more importantly, high stability, which thus has pinned great expectation as more promising photoelectrodes for PEC applications. 2,5-Dimethoxy-2,5-dihydrofuran (DMDF) has been considered a key intermediate for producing pyridines, pyridazines, pyrroles, benzenoid compounds, and coumarin analogs [27] , [28] , [29] , [30] . In its traditional chemical synthetic method, a large amount of bromine is employed as an oxidant, the mass usage of which raises issues of environmental pollution [29] . As an alternative approach to produce DMDF, electrochemical oxidation of furan can be mildly implemented in NH 4 Br alcoholic solution. In 2017, Sayama and co-worker provided another more direct approach based on a PEC system using BiVO 4 /WO 3 as a photoanode with a Br + /Br − mediator under visible light irradiation [30] . PEC synthesis has been found to significantly lower the required applied potential; however, the resulting photocurrent density is slightly unsatisfactory (<0.55 mA cm −2 ). Currently, it is reasonable to expect that halide perovskite SCTFs could deliver advanced PEC performance towards DMDF production, considering their remarkable photoelectric properties. However, the utilization of perovskite-based PEC cells for organic synthesis remains unexplored. Herein, methylammonium lead bromide MAPbBr 3 SCTF grown on a conductive FTO glass substrate is demonstrated as an efficient photoanode in a PEC cell to afford a high turnover rate for artificial photosynthesis of DMDF from furan. The surface is the most vulnerable to defects and passivation of single-crystal surface defects is the most important task. The subsequent deposition of Al 2 O 3 and Ti overlayers significantly promoted the operating stability and photocatalytic activity of MAPbBr 3 SCTFs. As an encouraging result, the highest photocurrent of 7.8 mA cm −2 (0.8 V vs. Ag/AgCl) is achieved for MAPbBr 3 SCTF/Al 2 O 3 /Ti. Such work paves the way for the future design of high-performance perovskite SCTF-based solar-driven photosynthesis systems. PEC characterizations of MAPbBr 3 SCTF and PCTF MAPbBr 3 SCTFs were grown in situ on an FTO/TiO 2 substrate through our previously reported space-limited crystallization method with some modifications [31] , [32] . The as-prepared MAPbBr 3 SCTF exhibits a smooth and pinhole-free surface with a lateral size of 11.5 mm × 7.6 mm and a film thickness of approximately 14 µm (Fig. 1 a, b and Supplementary Fig. 1a ). In contrast, a 300-nm-thick MAPbBr 3 PCTF prepared by spin-coating (Fig. 1c and Supplementary Fig. 1b ) is composed of small crystals accompanied by abundant sharp grain boundaries (Fig. 1d ). The configuration of the PEC cell system is depicted in Fig. 1e , where MAPbBr 3 SCTF (or PCTF) on an FTO/TiO 2 substrate and a Br − /Br + redox couple in an acetonitrile/methanol mixed solution function as the photoanode and electrolyte, respectively. Ultraviolet photoelectron spectra (UPS, Supplementary Fig. 2a , b) show that the valence band maximum (VBM) of the MAPbBr 3 SCTF is approximately 1.45 V vs. SHE, capable of bromine oxidation (0.7 V vs. SHE, Supplementary Fig. 2c ) [28] . Upon light excitation, the Br − in the electrolyte will be oxidized into Br + species by photogenerated holes, which then serve as oxidizing reagents to transform furan into DMDF. The resultant saturated photocurrent densities of MAPbBr 3 PCTF and SCTF are 0.7 and 1.2 mA cm −2 at 0.20 V vs. Ag/AgCl (Fig. 1f ), respectively. Such a 70% enhancement in photocurrent density for MAPbBr 3 SCTF is mainly ascribed to its high crystallinity, high charge mobility and low trap density [31] . In addition, it can be clearly seen that the photocurrent density of the MAPbBr 3 PCTF PEC cell decreases rapidly within ~3 min, while that of the MAPbBr 3 SCTF retains 54% of the initial value even after 30 min (Fig. 1g ). This phenomenon is further supported by the stability of the materials in acetonitrile/methanol electrolyte (Supplementary Fig. 3 ). MAPbBr 3 PCTF decomposed within 25 min, while MAPbBr 3 SCTFs exhibit negligible degradation even after 20 h, further demonstrating the better stability of SCTFs. The diffusion length of MAPbBr 3 SCTF (5.6 µm) [31] is much higher than that of perovskite-based thin films (0.33 µm) [33] . Electric fields can help carriers migrate from a 14 µm thick single crystal to the surface and then participate in chemical reactions. On the premise of ensuring light absorption, further reducing the thickness of single crystal film is beneficial for shortening the carrier transmission distance and further improving the PEC performance. However, it is still challenging to control the perovskite single crystal films with large size and several microns thickness. In terms of influence of thickness on stability of perovskite film, thicker films tend to exhibit better stability (Supplementary Fig. 4 ). However, grain boundaries in PCTF have also been widely proven to primarily bear the brunt of perovskite degradation due to massively distributed trap states [34] . Therefore, the stability of the SCTF-based PEC cell can be mainly ascribed to the advantages of being few defect states. Fig. 1: Comparison of MAPbBr 3 SCTF with PCTF. Optical microscopy and SEM images of MAPbBr 3 SCTF ( a , b ) and PCTF ( c , d ). e Schematic configuration of the proposed working principle of MAPbBr 3 SCTF-based (or PCTF-based) PEC cells. f Linear sweep voltammetry (LSV) of MAPbBr 3 SCTF-based and PCTF-based photoelectrodes. g Chronoamperometric trace of MAPbBr 3 SCTF-based and PCTF-based photoelectrodes recorded at an applied potential of 0.2 V vs. Ag/AgCl. Full size image Investigation of the Al 2 O 3 passivation effect for MAPbBr 3 SCTFs Halide perovskite materials have been widely proven to have a low trap formation energy and reconfigurable surface lattice [35] , [36] , and therefore, surface trap states are easily formed as charge carrier recombination centers [37] . Herein, we deposit an ultrathin Al 2 O 3 layer onto a MAPbBr 3 SCTF through atomic layer deposition (ALD) to further boost the PEC performance by reducing the amounts of surface trap states (see section “Experimental details” in the “Methods” section). The presence of Al 2 O 3 is first verified by the additional Al 2 p peak at 74.8 eV in the X-ray photoelectron spectroscopy (XPS) spectra (Fig. 2a ). Furthermore, characteristic signals of Al–CH 3 , (OH)–Al=O and Al–O–Al species are observed at 1256, 1080, and 888 cm −1 in the Fourier transform infrared (FTIR) spectra after ALD treatment, again proving the existence of Al 2 O 3 (Supplementary Fig. 5a ). During the process of ALD deposition of Al 2 O 3 , TMA reacts with CH 3 NH 3 + of MAPbBr 3 and results in CH 3 NH 2 release accompanied by the formation of Br 3 Pb–Al(CH 3 )–PbBr 3 intermediates (Fig. 2d ) [38] , which further react with O 2 to produce Al 2 O 3 . Further insight into the chemical modification on the perovskite surface was provided by comparing the surface XPS spectra of N 1 s , Pb 4 f , and Br 3 d before and after Al 2 O 3 deposition (Fig. 2 a– c ). The intensity of the N 1 s peak is significantly weakened due to CH 3 NH 2 release. Furthermore, both Pb 4 f 7/2 and Pb 4 f 5/2 peaks (Fig. 2c ) shift to lower binding energy values by 0.37 eV after the ALD process because of the Pb-rich surface defects bonded with adsorbed oxygen [39] , [40] , which can additively suppress nonradiative recombination on the perovskite surface. The surface microstructure of the MAPbBr 3 SCTF is well retained after Al 2 O 3 deposition, as revealed from the scanning electron microscopy (SEM) image (Supplementary Fig. 5b ). Identical X-ray diffraction (XRD) patterns are observed in MAPbBr 3 SCTF and MAPbBr 3 SCTF/Al 2 O 3 with the same growth orientation along the (h00) crystal plane, which not only reveals that the crystal phase of perovskite is well preserved during the ALD process, but also implies that the deposited Al 2 O 3 is thin/amorphous (Supplementary Fig. 6 ). Fig. 2: Al 2 O 3 passivation effect investigation. XPS spectra of pristine MAPbBr 3 SCTF and MAPbBr 3 SCTF/Al 2 O 3 : Al 2 p and Br 3 d ( a ), N 1 s ( b ), and Pb 4 f ( c ). d Proposed passivation mechanism of Al 2 O 3 on the MAPbBr 3 SCTF surface. e PEC behavior of MAPbBr 3 SCTF/Al 2 O 3 -based photoelectrodes as a function of Al 2 O 3 deposition thickness. Al 2 O 3 -thickness-dependent steady-state photoluminescence (PL) spectra ( f ) and time-resolved PL decay curves ( g ). Full size image A batch of MAPbBr 3 SCTF/Al 2 O 3 (0, 1, 5, and 10 nm) were fabricated by adjusting the ALD deposition cycles to unlock the effect of the Al 2 O 3 layer on the PEC performance. Al 2 O 3 thickness is achieved by controlling the number of ALD deposition cycles. Approximately 0.1 nm of aluminum oxide was deposited per cycle (for instance, 50 cycles, namely 5 nm). As shown in Fig. 2e , the saturated photoanode current density of the pristine MAPbBr 3 SC film is ~1.2 mA cm −2 at 0.4 V vs. Ag/AgCl (0.53 V vs. SHE, Supplementary Fig. 7 ), which gradually increases with thickening Al 2 O 3 and reaches a maximum value of 5.5 mA cm −2 at 5 nm of Al 2 O 3 . The enhanced PEC performance affirms that the ultrathin Al 2 O 3 layer would not hinder photogenerated holes injection from perovskite to the electrolyte due to charge tunnelling. Comparing with pristine MAPbBr 3 SC, coating a thin Al 2 O 3 overlayer with a thickness of 1–10 nm resulted in slight overpotential increasement. This is because that deposited Al 2 O 3 can isolate the photoelectrode from the electrolyte, therefore the photocorrosion phenomenon of MAPbBr 3 SC being oxidized can be effectively suppressed. Meanwhile, with the increase of the thickness of Al 2 O 3 overlayer, the passivation of effect of MAPbBr 3 SC surface is more sufficient, so that the thicker 10 nm Al 2 O 3 can reduce the overpotential comparing to the thinner Al 2 O 3 (1 and 5 nm). The specific passivation mechanism will be discussed later. However, further thickening of the Al 2 O 3 layer (e.g., 10 nm) attenuated the photoanodic current density, probably due to the aggrandized charge transport resistance as a result of its intrinsic insulating properties. The PEC performance of MAPbBr 3 SCTF/Al 2 O 3 (5 nm) is ~10 times higher than that of a previously reported BiVO 4 /WO 3 photoanode with a maximum photocurrent of 0.55 mA cm −2 at 0.5 V vs. SHE) [28] . We have also investigated the influence of Al 2 O 3 thickness on the stability. The stability of the electrode gradually improved with the increase of the thickness of Al 2 O 3 from 0 to 10 nm (Supplementary Fig. 8 ), since the deposited Al 2 O 3 can isolate photoelectrode from the electrolyte. To identify the underlying reason for the increased PEC performance after coupling with an ultrathin Al 2 O 3 layer, the optical properties of MAPbBr 3 SCTF/Al 2 O 3 were investigated. As shown in Fig. 2f , the PL emission intensity of the MAPbBr 3 SCTF is significantly amplified after depositing 1-nm-thick Al 2 O 3 , and is further increased upon thickening of the Al 2 O 3 layer to 5 and 10 nm. Time-resolved PL (TRPL) decay plots at the emission maximum (Fig. 2g ) also demonstrate that all MAPbBr 3 SCTF/Al 2 O 3 samples decay sluggishly compared with pristine MAPbBr 3 SCTF. 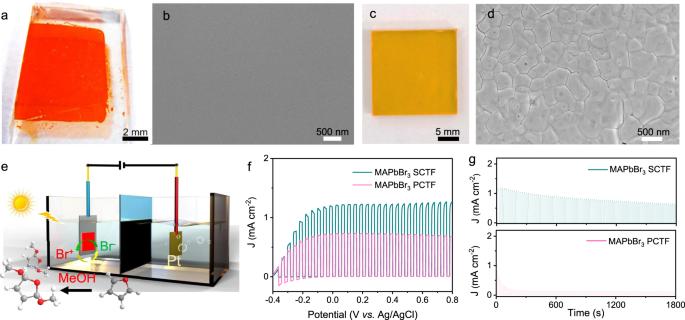Fig. 1: Comparison of MAPbBr3SCTF with PCTF. Optical microscopy and SEM images of MAPbBr3SCTF (a,b) and PCTF (c,d).eSchematic configuration of the proposed working principle of MAPbBr3SCTF-based (or PCTF-based) PEC cells.fLinear sweep voltammetry (LSV) of MAPbBr3SCTF-based and PCTF-based photoelectrodes.gChronoamperometric trace of MAPbBr3SCTF-based and PCTF-based photoelectrodes recorded at an applied potential of 0.2 V vs. Ag/AgCl. Specifically, the fitted average PL decay time of MAPbBr 3 SCTF/Al 2 O 3 (5 nm) is twofold longer than that of pristine MAPbBr 3 SCTF (Supplementary Table 1 ). 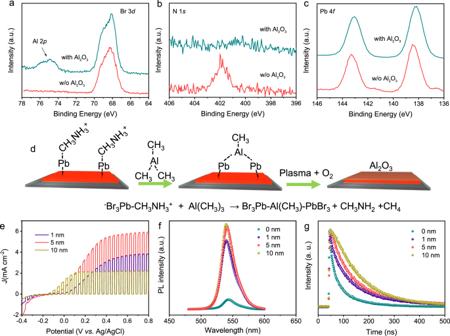Fig. 2: Al2O3passivation effect investigation. XPS spectra of pristine MAPbBr3SCTF and MAPbBr3SCTF/Al2O3: Al 2pand Br 3d(a), N 1s(b), and Pb 4f(c).dProposed passivation mechanism of Al2O3on the MAPbBr3SCTF surface.ePEC behavior of MAPbBr3SCTF/Al2O3-based photoelectrodes as a function of Al2O3deposition thickness. Al2O3-thickness-dependent steady-state photoluminescence (PL) spectra (f) and time-resolved PL decay curves (g). This enhanced PL intensity and prolonged PL lifetime can be ascribed to the suppression of nonradiative recombination of electron-hole pairs in MAPbBr 3 SCTF/Al 2 O 3 . In addition, spatial and temporal imaging PL emission was monitored with a sample size of 100 µm × 100 µm. 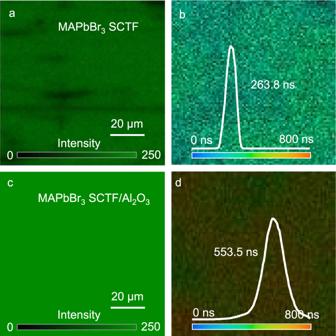Fig. 3: Fluorescence spectroscopic measurements. Confocal fluorescence intensity images (left) and fluorescence lifetime imaging microscopy (FLIM) images (right) of pristine MAPbBr3SCTF (a,b) and MAPbBr3SCTF/Al2O3(c,d). Figure 3a , c show confocal fluorescence images of pristine MAPbBr 3 SCTF and MAPbBr 3 SCTF/Al 2 O 3 (5 nm). Apparently, greater brightness is observed for MAPbBr 3 SCTF/Al 2 O 3 , corresponding to stronger PL emission intensity. More importantly, brightness contrast appears with apparent darker spots in the images of pristine MAPbBr 3 SCTF, but these spots are well dispelled after Al 2 O 3 deposition, thus affording a uniform PL emission image (Fig. 3c ). These darker spots on MAPbBr 3 SCTF could be assigned to the region with higher surface trap-state density, and thus with active nonradiative charge carrier recombination [41] . Agreeing well with the TRPL test, fluorescence lifetime imaging microscopy (FLIM, Fig. 3b, d ) data suggest a longer average PL lifetime for MAPbBr 3 SCTF/Al 2 O 3 (553.5 ns) than for pristine MAPbBr 3 SCTF (263.8 ns). These results strongly affirm the passivation role of Al 2 O 3 , which effectively suppresses the trap states on the perovskite surface [42] . Fig. 3: Fluorescence spectroscopic measurements. Confocal fluorescence intensity images (left) and fluorescence lifetime imaging microscopy (FLIM) images (right) of pristine MAPbBr 3 SCTF ( a , b ) and MAPbBr 3 SCTF/Al 2 O 3 ( c , d ). Full size image Different from the PL tests, transient reflection (TR) spectroscopy (Fig. 4a ) can solely monitor the surface luminous and nonluminous species and provide detailed insight into the surface charge carrier dynamics, avoiding interferential signals from the bulk [37] , [43] . Both pristine MAPbBr 3 SCTF and MAPbBr 3 SCTF/Al 2 O 3 feature a bandgap of 2.36 eV, corresponding to a UV–Vis absorption onset at 525 nm (Supplementary Fig. 9 ). Therefore, a 400 nm laser pulse with corresponding penetration depths of 80 nm was employed to excite only MAPbBr 3 [44] , and broadband continuum white light in the range of 450–700 nm was used as the probe pulse to monitor the reflection difference. 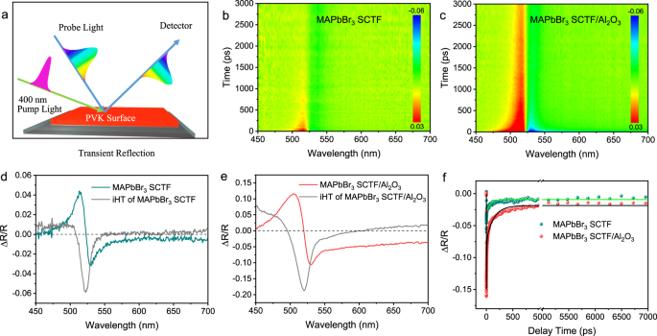Fig. 4: Transient reflection spectroscopic measurements. aDiagram of transient reflection (TR); TR spectra pseudocolour images, and TR spectra recorded at a delay time of 5 ps of pristine MAPbBr3SCTF (b,d) and MAPbBr3SCTF/Al2O3(c,e). Kinetic fit of the data of these two SCTFs (f). Figure 4b , c show the pseudocolour TR spectra of pristine MAPbBr 3 SCTF and MAPbBr 3 SCTF/Al 2 O 3 , both characterized by an intense signal at approximately 520 nm. Accordingly, transient TR profiles recorded at a delay time of 5 ps also show a typical antisymmetric peak centred at 520 nm (Fig. 4d , e). To clearly reveal the transient absorption (TA) difference upon light excitation, the inverse Hilbert transform (iHT) was performed according to the Kramers–Kronig relationship [45] . As displayed in Fig. 4d , e, the resultant TA curves after iHT exhibit a ground state bleaching peak centred at ~520 nm, agreeing well with the absorption onset. Due to the restricted time window (≤7 ns) for the TR tests, the decay dynamics are mainly derived from the diffusion and recombination processes of surface photo-induced charge carriers [46] . The decay kinetics probed at 520 nm (Fig. 4f ) were analysed and interpreted and show a very sluggish decay for MAPbBr 3 SCTF/Al 2 O 3 compared to that of the pristine MAPbBr 3 SCTF (141 ps vs. 70 ps) due to the retardative surface trap-assisted recombination afforded by the ultrathin Al 2 O 3 layer. Fig. 4: Transient reflection spectroscopic measurements. a Diagram of transient reflection (TR); TR spectra pseudocolour images, and TR spectra recorded at a delay time of 5 ps of pristine MAPbBr 3 SCTF ( b , d ) and MAPbBr 3 SCTF/Al 2 O 3 ( c , e ). Kinetic fit of the data of these two SCTFs ( f ). 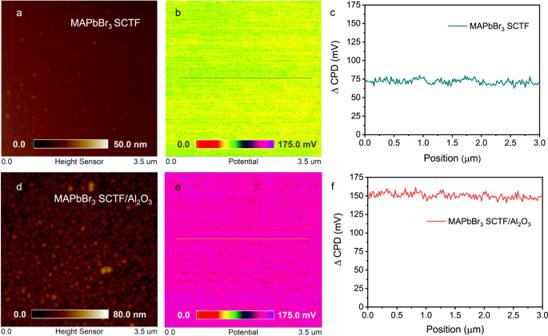Fig. 5: Kelvin probe force microscopy. AFM topography images, KPFM images and△CPD profiles (subtracting the potential in the dark from that under light irradiation) of pristine MAPbBr3SC film (a–c) and MAPbBr3SCTF/Al2O3(d–f). Full size image To further investigate the underlying effect of the Al 2 O 3 layer on the electrical properties of the MAPbBr 3 SCTF, Kelvin probe force microscopy (KPFM) was performed to probe the spatial charge transfer and separation on the perovskite. After subjection to the ALD 5 nm procedure, the MAPbBr 3 SCTF surface appears slightly rougher with an increase in the root-mean-square value from 0.7 to 5.7 nm (Fig. 5a , d). Continuously distributed nanosized particles can be clearly observed in Fig. 5d , further corroborating that an ultrathin compact Al 2 O 3 layer was uniformly deposited onto the MAPbBr 3 SCTF, which is associated with island growth mechanism during ALD deposition of Al 2 O 3 [38] . The KPFM images and the corresponding line profiles of the surface photovoltage (SPV) difference are displayed in Fig. 5b, c, e, f . MAPbBr 3 behaves as an n -type semiconductor according to UPS analysis, thus resulting in a space charge layer at the surface with an inherent electric field direction from the interior towards the surface [47] . The positive SPV values of MAPbBr 3 SCTF and MAPbBr 3 SCTF/Al 2 O 3 indicated the photoinduced holes could transfer from the interior to surface of the sample. The SPV value of MAPbBr 3 SCTF/Al 2 O 3 is approximately 150 mV, twice higher than that of pristine MAPbBr 3 PCTF (75 mV), indicating richer density of holes accumulated onto the surface, which is beneficial for enhancing the PEC performance. Fig. 5: Kelvin probe force microscopy. AFM topography images, KPFM images and △ CPD profiles (subtracting the potential in the dark from that under light irradiation) of pristine MAPbBr 3 SC film ( a – c ) and MAPbBr 3 SCTF/Al 2 O 3 ( d – f ). Full size image Investigation of the Ti layer effect on the PEC performance of MAPbBr 3 SCTFs The above experimental results reveal that the Al 2 O 3 passivation layer significantly enhances the PEC performance and the stability of the photoelectrode to some extent. However, due to its ultrathin thickness, long-term PEC stability is still challenging to maintain. Conductive overlayers have been widely proven to enhance the operating stability and even catalytic activity of semiconductor materials [8] , [13] . Thus, a 145-nm-thick Ti layer with a particle size of approximately 30 nm (Supplementary Fig. 10 ) was introduced onto MAPbBr 3 SCTF/Al 2 O 3 as a protective layer to avert direct interaction with the electrolyte. The MAPbBr 3 SCTF/Al 2 O 3 /Ti shows almost the same XRD pattern as MAPbBr 3 (Supplementary Fig. 11a ). The reasons beyond the failure to observe the characteristic XRD pattern of Ti layer probably can be concluded as follows: (a) the high crystallinity of perovskite single crystal leads to its diffraction signals completely overwhelms the Ti signals; (b) amorphous nature of the deposited Ti layer. In order to find out the underlying reasons, we have tried to deposit Ti layer on the surface of quartz. The XRD results (Supplementary Fig. 11b ) show that there are two new phases, which can be assigned to the Ti (PDF#01-074-7075) and rutile TiO 2 (PDF#04-008-7856) with low crystallinity. The formation of TiO 2 is ascribed to the oxidation of titanium by residual oxygen in the system during the evaporation process [48] . XPS spectrum (Supplementary Fig. 12 ) reveals that metallic Ti 0+ (at 454.1 and 460.2 eV), Ti 3+ (at 456.9 and 462.4 eV) and Ti 4+ (at 458.7 and 464.4 eV) species are present, implying a TiO x -rich surface [49] . 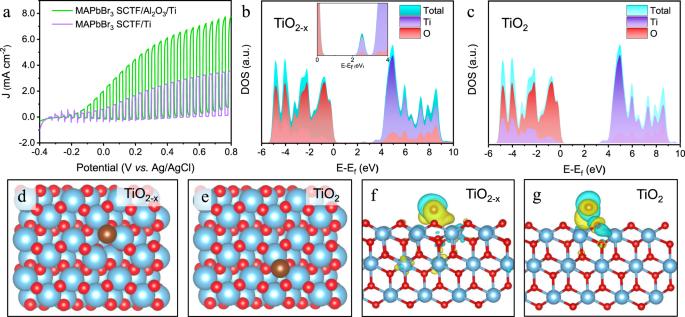Fig. 6: Ti layer effect on the PEC performance. aPEC behaviors of MAPbBr3SCTF/Ti-based and MAPbBr3SCTF/Al2O3/Ti-based photoelectrodes. The projected DOS ofbTiO2−xandcTiO2. DFT-calculated adsorption of Br on the surfaces ofdTiO2−xandeTiO2.f,gCorresponding electron density difference, where yellow indicates a gain of electrons and cyan indicates loss of electrons. Figure 6a displays the current-potential curves of the MAPbBr 3 SCTF/Al 2 O 3 /Ti-based PEC cell under chopped illumination. After incorporating the Ti layer on the MAPbBr 3 SCTF/Al 2 O 3 photoanode, the onset potential (~0.2 mA cm −2 ) [50] was negatively shifted by 120 mV. The photocurrent was saturated for MAPbBr 3 /Al 2 O 3 (5 nm) at 0.4 V vs. Ag/AgCl with 5.5 mA cm −2 . In contrast, the photocurrent is not saturated for MAPbBr 3 SCTF/Al 2 O 3 /Ti throughout all the test voltages from −0.4 to 0.8 V, reaching 7.8 mA cm −2 at 0.8 V vs. Ag/AgCl. To confirm the catalytic activity of Ti layer, the electrochemical behavior of FTO/Ti and FTO was also studied (Supplementary Fig. 13 ). Compared with the weak anodizing current of the FTO electrode, the FTO/Ti electrode exhibited remarkable electrocatalytic activity towards bromine oxidation with a near-zero overpotential and an onset potential of 0.73 V vs. SHE (0.60 V vs. Ag/AgCl). This result indicates that holes can easily be injected into the electrolyte and immediately participate in the chemical reaction due to the co-catalyst function of the Ti layer. Fig. 6: Ti layer effect on the PEC performance. a PEC behaviors of MAPbBr 3 SCTF/Ti-based and MAPbBr 3 SCTF/Al 2 O 3 /Ti-based photoelectrodes. The projected DOS of b TiO 2−x and c TiO 2 . DFT-calculated adsorption of Br on the surfaces of d TiO 2−x and e TiO 2 . f , g Corresponding electron density difference, where yellow indicates a gain of electrons and cyan indicates loss of electrons. Full size image Density functional theory (DFT) calculations were conducted to shed light on the impact of Ti species on the electronic properties of the materials [51] . As shown in Supplementary Fig. 14 , the calculated density of state (DOS) of Ti is continuous owing to its intrinsic metallic nature. Figure 6b , c illustrate that Ti 3+ produces a higher density of oxygen vacancies and rearranges the band structure. The interaction between the Br atom and the three-atomic-layer p(3x) surface was probed (Fig. 6d , e). The calculated Br adsorption energy is more negative for TiO 2 (−3.61 eV) than for TiO 2−x (−0.57 eV), implying that TiO 2−x has more potential as a Br oxidation catalyst. Upon adsorption, Br atoms suffer from charge redistribution and form chemical bonds with Ti atoms. The length of the Ti–Br bond on the TiO 2−x surface (2.59 Å) is estimated to be shorter than that on TiO 2 (2.67 Å), agreeing well with its advantageous Br adsorption owing to the low-coordinated oxygen surface. The charge difference analysis in Fig. 6f , g displays a more significant charge transfer on the TiO 2−x surface than on the TiO 2 surface. Based on Mulliken charge analysis, the Br atom is −0.26|e| on TiO 2−x but only −0.06|e| on TiO 2 . A similar trend has been observed based on Bader charge analysis, i.e., −0.54|e| on TiO 2−x and −0.26|e| on TiO 2 . The increased electron cloud density of Br favours the harvesting of holes during the subsequent oxidation process. Similar phenomena have also been observed in defect-rich TiO 2 , where the oxygen vacancies and Ti 3+ ions facilitate more efficient charge transfer [52] and serve as an intrinsic active species to increase the electrochemical [53] , photocatalytic, and PEC activities [54] . The current calculation results are consistent with the hypothesis that the introduction of catalytic active sites on the surface of the photoelectrode promotes the further improvement of PEC performance. In addition to affording superior PEC performance, Ti overlayer can also protect the internal Al 2 O 3 layer and perovskite layer. In order to further mitigate the influence of the electrolyte penetration from the edge, silicone sealant (Kafuter K-705) is used to encapsulate the edge of electrode. The resulted photoelectrode exhibited impressive stability for DMDF evolution, as displayed in Supplementary Fig. 15 . The Br-mediated photogeneration of DMDF was carried out at 0.2 V vs. Ag/AgCl, which is lower than the potential required to initiate the electrochemical oxidation of bromine. The photocurrent density is well maintained even after 6 h of continual electrolysis at 0.2 V. The formation of DMDF is confirmed via mass spectrometry (Supplementary Fig. 16 ), and the Faraday efficiency is calculated to be as high as 93%, further promising its infinite potential as an effective and stable photoelectrode. In summary, a MAPbBr 3 SCTF-based photoanode could drive the conversion of furan to DMDF has been demonstrated. Combined investigations with FLIM and TR as well as KPFM characterizations demonstrated that an ultrathin Al 2 O 3 layer effectively suppressed trap-assisted nonradiative charge recombination, resulting in a doubled surface charge carrier lifetime. Furthermore, the subsequent deposited Ti layer not only stabilized the MAPbBr 3 SCTF by isolating perovskite from the electrolyte but also facilitated the bromine-mediated oxidation of furan owing to the Ti 3+ catalytic active site. As a result, the highest photocurrent of 7.8 mA cm −2 at 0.8 V vs. Ag/AgCl was realized for the MAPbBr 3 SCTF/Al 2 O 3 /Ti photoanode. The photoanode retained remarkable stability for more than 6 h under chopped light illumination. Considering the lead-related-toxic issues [55] , [56] , stable lead-free perovskite SCTFs should deserve more future research focus towards environment-friendly and efficient photocatalysts, whose application will be potentially expanded to currently still challenging biomass conversion and organic synthesis reactions in the near future. Synthesis of methylammonium bromide (MABr) A mixture of methylamine solution (30–33 wt% in methanol, Aladdin) and hydrobromic acid (48 wt% in water, Aladdin) with a molar ratio of 1:1.5 was stirred in an ice-water bath for 2 h. After that, MABr powder was precipitated by rotary evaporating the solvent at 50 °C and then purified by recrystallization. The collected MABr powder was dried in a vacuum oven for 24 h. Fabrication of MAPbBr 3 single-crystal thin films (SCTFs) MAPbBr 3 SCTFs were grown onto TiO 2 -coated FTO glass substrates according to our previously reported method [31] , [32] . First, FTO glass substrates (7 Ω square −1 , Nipponsheet Glass) were sequentially cleaned by ultrasonication in detergent water, alcohol, and acetone for 30 min per step. A compact TiO 2 layer was subsequently deposited on the cleaned FTO glass via spin-coating of a TiO 2 colloidal solution at 4 k rpm for 30 s, followed by an annealing process at 500 °C for 30 min. The annealed TiO 2 -coated FTO substrate was further immersed into a 0.04 M TiCl 4 solution at 70 °C for 30 min before a secondary annealing process at 500 °C. A space-limited model was assembled by sandwiching a thin polytetrafluoroethylene rectangular ring frame (20 μm in thickness) into two pieces of TiO 2 -coated FTO glasses. Then, the MAPbBr 3 precursor solution, prepared by dissolving equimolar PbBr 2 and MABr in DMF, was circulated into the limited space between the two substrates by a peristaltic pump (BT100-2J, Longer Pump). Note that the bottom FTO glass was drilled with two holes to facilitate the circulation of the perovskite precursor solution. The middle part of the model was locally heated to 95 °C for crystallization and then maintained at 80 °C for crystal growth. After ~72 h, the two FTO glasses were separated, with MAPbBr 3 SCTFs grown in situ on the conductive substrate. The precipitated polycrystals were removed by γ-butyrolactone, and the residual solution was cleaned and removed by vacuum drying. Fabrication of MAPbBr 3 PCTF Equimolar MABr and PbBr 2 were dissolved in DMF/DMSO (3:1, v–v) at a concentration of 1.2 M. An appropriate amount of perovskite precursor solution was spin-coated onto the substrate with a ramp rate of 3000 rpm, and 200 µL of chlorobenzene was dropped onto the spinning substrate 10 s after the spin-coating began. The obtained film was annealed at 120 °C for 10 min. Fabrication of MAPbBr 3 SCTF/Al 2 O 3 /Ti An ultrathin aluminum oxide layer was grown on the surface of MAPbBr 3 SCTF by an atomic layer deposition (ALD) machine (ALD-SC6-PE, Syskey) with TMA and plasma oxygen as the element sources. In each ALD cycle, TMA was dosed into the chamber for 80 ms and purged out by Ar gas for 8 s, followed by dosing plasma O 2 into the chamber for 3 s and purging out by Ar gas for 8 s. Approximately 0.1 nm of aluminum oxide was deposited per cycle. The ALD chamber was kept at a substrate temperature of 80 °C to achieve effective deposition of Al 2 O 3 . Another thin layer of Ti was further deposited on the aluminum oxide layer by the thermal evaporation deposition method (SKY Technology Development). Characterizations XRD patterns were collected on a Rigaku Miniflex 600 X-ray diffractometer with Cu K α radiation ( λ = 1.5418 Å). X-ray photoelectron spectroscopy (XPS) was performed by means of a Thermo-VG Scientific ESCALAB 250 X-ray photoelectron spectrometer. The cross-sectional surface morphology and film thickness were examined by high-resolution field emission scanning electron microscopy (FE-SEM, Gemini 500). Atomic force microscopy (AFM) and scanning KPFM measurements were performed on a Bruker Dimension Fast Scan AFM system. UV–Vis absorption was obtained on an ultraviolet–visible spectrophotometer (Shimadzu UV-3600). Photoluminescence (PL) spectra were obtained on a fluorescence spectrophotometer (Edinburgh FLS980) with an excitation wavelength of 406 nm. Confocal fluorescence images and fluorescence-lifetime imaging microscopy (FLIM) images were recorded on a Zeiss LSM880 NLO microscope with an excitation wavelength at 405 nm. Transient reflectance spectra were measured on a Helios (Ultrafast Systems LLC) pump-probe setup in reflection mode. The pump beam at 400 nm was generated in a collinear optical parametric amplifier (OPerA Solo, Coherent) pumped by 800 nm fundamental pulses (100 fs, 1 kHz repetition rate, Astrella-Tunable-V-F-1k, Coherent). A sapphire crystal was used to generate a broad white light continuum probe spectrum. The TR signal changes were recorded in the visible region from 450 to 700 nm. DFT calculations DFT calculations were carried out by means of the CP2K package [57] . The PBE functional [58] with Grimme D3 correction [59] and Goedecker-Teter-Hutter (GTH) pseudopotentials [60] , [61] and DZVPMOLOPT-GTH basis sets [62] were utilized to describe the system and the molecules, respectively. Unrestricted Kohn–Sham DFT was performed as the electronic structure method in the framework of the Gaussian and plane waves method [62] , [63] . A plane-wave energy cut-off of 500 Ry was employed. The adsorption energy ( E b ) is defined as: 
    E_b = E_Br/sur - 1/2E_Br_2(g) - E_sur,
 (1) where E Br/sur , \({{E}}_{{\mathrm{Br}}_2}\) , and E sur are the surface Br adsorption energy and the individual electron density of the molecule and surface, respectively. The charge density difference (Δ ρ ) is defined as 
    Δρ = ρ _Br/sur - ρ _Br - ρ _sur,
 (2) where ρ Br/sur , ρ Br , and ρ sur are the electron density of surface-adsorbed Br and the individual electron density of Br and surface, respectively. Photoelectrochemical (PEC) measurements PEC performance was measured on an electrochemical workstation (CHI660E, CH Instruments) at room temperature. A conventional three-electrode system with a Pt mesh as a counter electrode and Ag/AgCl (sat KCl) as a reference electrode was adopted. To prevent dissolution and decomposition of perovskite, excessive MABr (2.02 g) was added to a mixed solution of anhydrous acetonitrile (45 mL) and anhydrous methanol (5 mL) as an anolyte. To prepare the target product of 2,5-dihydro-2,5-dimethoxyfuran, an additional 2.5 mL of furan (Innochem) was added. For the catholyte, 1-butyl-1-methylpyrrolidinium bis(trifluoromethylsulfonyl)imide (3.47 g, 99%, Shanghai Cheng Jie Chemical) and deionized water (0.5 mL) were added to anhydrous acetonitrile (50 mL). The linear sweep voltammogram (LSV) curves were measured at a scanning rate of 10 mV s −1 from −0.4 V to 0.8 V vs. Ag/AgCl under simulated solar illumination (Zolix, Gloria-X150A, 100 mW cm −2 , AM 1.5G filtered, calibrated with a standard Si solar cell). The light on/off was regulated by the light chopping equipment (Perfect Light, PFS40A). After the photoelectrocatalysis test, 2 mL H 2 O was added into 1 mL of anode electrolyte and the solution was extracted with 0.5 mL ethyl acetate. The 2,5-dihydro-2,5-dimethoxyfuran in the top organic layer was quantitatively analyzed by gas chromatography using commercial 2,5-dihydro-2,5-dimethoxyfuran (TCI Shanghai) diluted with ethyl acetate as an external standard.